N-cadherin regulates spatially polarized signals through distinct p120ctn and β-catenin-dependent signalling pathways The spatial distribution of molecular signals within cells is crucial for cellular functions. Here, as a model to study the polarized spatial distribution of molecular activities, we used cells on micropatterned strips of fibronectin with one end free and the other end contacting a neighbouring cell. Phosphoinositide 3-kinase and the small GTPase Rac display greater activity at the free end, whereas myosin II light chain and actin filaments are enriched near the intercellular junction. Phosphoinositide 3-kinase and Rac polarization depend specifically on the N-cadherin–p120catenin complex, whereas myosin II light chain and actin filament polarization depend on the N-cadherin–β-catenin complex. Integrins promote high phosphoinositide 3-kinase/Rac activities at the free end, and the N-cadherin–p120catenin complex excludes integrin α5 at the junctions to suppress local phosphoinositide 3-kinase and Rac activity. We hence conclude that N-cadherin couples with distinct effectors to polarize phosphoinositide 3-kinase/Rac and myosin II light chain/actin filaments in migrating cells. Directional and collective cell migration in vivo, such as endothelial, immune and fibroblast cells migrating towards ischaemic tissues and wounds, is crucial for tissue remodelling and organism survival [1] . Efficient migration requires cell polarization, with distinct activities at the leading edge and trailing regions [2] . The major driving forces in migrating single cells are from Rac-dependent actin polymerization at the leading edge and Rho-dependent acto-myosin contraction at the rear. Multiple mechanisms contribute to Rac polarization and the subsequent actin polymerization at the leading edge [2] , [3] . Phosphoinositide 3-kinase (PI3K) and its lipid product phosphatidyl inositol-3,4,5-triphosphate are concentrated at the leading edge and recruit Rac guanine-nucleotide exchange factors to the plasma membrane to activate Rac [4] , [5] . Rac in turn can regulate PI3K activity via both direct binding [6] and through downstream pathways, including superoxide [5] to establish a positive feedback loop [1] . A second positive feedback loop involves integrins, which also activate Rac at the leading edge through multiple mechanisms [1] , [7] , [8] , while Rac promotes formation of new adhesion and localization of high-affinity integrins at the leading edge [9] . At the rear, Rho controls the assembly of acto-myosin to generate contractile force and promote detachment of the cell tail [2] . The acto-myosin machinery consists of myosin II and actin stress fibres, regulated by the coordination of myosin light chain (MLC) phosphorylation and Ca 2+ at subcellular locations [10] . Despite these well-established mechanisms, it remains unclear how these processes are integrated temporally and spatially across the cell [2] . During collective migration in vivo , neighbouring cells remain connected through cadherin-mediated adherens junctions [11] . The intracellular tail of classic cadherins contains a juxtamembrane domain that binds p120catenin (p120ctn) and a C-terminal domain (CBD) that binds β-catenin [12] . P120ctn regulates cadherin stability [13] and Rho GTPases [14] , [15] . β-Catenin interacts with α-catenin, which can further couple to the actin cytoskeleton [12] . As such, connected to various signalling molecules, cadherins not only establish junctions but also regulate molecular polarity during migration. For example, N-cadherin is required for microtubule organizing centre orientation and directional migration of smooth muscle cells [16] . Similarly, E-cadherin mediates the effect of the mammalian Scribble (Scrib) polarity protein on directed migration of epithelial Madin–Darby canine kidney cells [17] . Elegant studies also indicate that N/E-cadherin can regulate cell polarization, including the polarized distribution of centrosome, lamellipodia dynamics and Rac1 activity [18] , [19] , [20] . However, the underlying mechanism by which cadherins coordinate and integrate the signalling network to regulate molecular polarity at subcellular levels remains poorly understood. Integrin-mediated cell–extracellular matrix (ECM) and cadherin-mediated cell–cell adhesions jointly regulate many cellular functions [21] . For example, integrin-dependent acto-myosin contraction physically ruptures E-cadherin-mediated cell–cell contacts during the scattering of epithelial cells [22] . Integrin-mediated activation of focal adhesion kinase and Src can affect the junction stability through the phosphorylation of cadherin/catenin [23] . Conversely, perturbing N-cadherin induces translocation of the non-receptor tyrosine kinase Fer from cadherin to the integrin complex and modulates the integrin-mediated adhesions [24] , [25] . E-cadherin can regulate Rap1 localization to suppress integrin function [26] . In contrast, TGFβ-induced loss of E-cadherin promotes the assembly of β1 integrin-dependent focal adhesions [26] , [27] . In response to mechanical shear stress stimulation, VE-cadherin, together with PECAM1 and VEGFR2, stimulate activation of integrin αvβ3 in endothelial cells [28] . In this study, we combine micropatterning technology with molecular biosensors for live cell imaging to study the coordination between cell–cell and cell–ECM adhesions in polarizing molecular signals. We found that N-cadherin-mediated adherens junctions promote activation of PI3K and Rac at the cell free end through p120ctn, which suppresses integrins near the junction. Additionally, N-cadherin promotes accumulation of MLC and actin filaments (AF) near the cell–cell junction through β-catenin. In summary, our results revealed a new molecular hierarchy in which N-cadherin regulates the subcellular distributions of different signalling molecules through distinct effectors. Distinct polarization patterns for PI3K/Rac and MLC/AF To study the role of cell–cell adhesions in coordinating signalling transduction at subcellular levels, we developed a cell model in which mouse embryonic fibroblasts (MEFs) were seeded on fibronectin (Fn)-coated strips with one end of the cell free and the other end contacting a neighbouring cell ( Supplementary Fig. S1a and Supplementary Movie 1 ). We first examined the subcellular distribution of PI3K and Rac activities, which regulate leading edge protrusion, and MLC and AF, which mediate cell contraction [2] . The GFP-fused PH domain of Akt (PH-Akt-GFP), which binds phosphatidyl inositol-3,4,5-triphosphate, was used to visualize the spatial distributions of PI3K activity [29] . PH-Akt-GFP fluorescence was diffusive in resting cells, but accumulated at the free end upon platelet-derived growth factor (PDGF) stimulation ( Fig. 1a and Supplementary Movie 2 upper panel). PDGF-induced polarization and translocation of PH-Akt-GFP started immediately after PDGF treatment and continued for about 10–20 min to reach stabilization of the polarity ( Supplementary Fig. S1b and Supplementary Movie 3 ). In contrast, the co-transfected fluorescent protein mCherry in these cells did not significantly translocate to the cell periphery following PDGF ( Fig. 1a ). Quantification of the fluorescence intensity distribution and GFP/mCherry ratio along the strip direction ( Supplementary Fig. S2 , quantification procedure detailed in Methods) confirmed the clear accumulation of PH-Akt-GFP but not mCherry at the free end upon PDGF stimulation ( Fig. 1b and Supplementary Fig. S3a ). 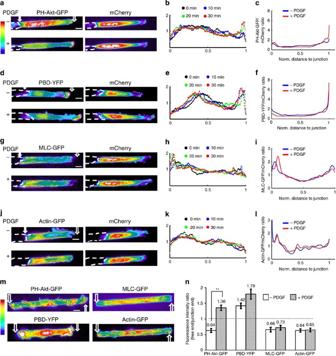Figure 1: The polarization of molecular signals. MEFs transfected with various fluorescent probes were seeded on Fn-coated strips (10 μm in width), with one end free and the other end contacting a neighbouring cell. The broken white lines represent the body contours of neighbouring cells physically contacting the cells of interest. The hollow and filled arrows on the images indicate the positions of the free and junction ends, respectively. (a–l) The fluorescence intensity distributions of mCherry together with (a–c) PH-Akt-GFP (n=4), (d–f) PBD-YFP (n=5), (g–i) MLC-GFP (n=4) or (j–l) actin-GFP (n=4) before and after PDGF stimulation. (a,d,gandj) The pseudo colour images represent the fluorescence intensity of different probes as indicated, with cold and hot colours representing low and high fluorescence intensities, respectively; (b,e,handk) The intensity distributions of indicated probes averaged along the strip direction before and after PDGF stimulation for various periods of time as indicated. (c,f,iandl) The averaged intensity ratios between the indicated probe and co-transfected mCherry along the strip direction before and after PDGF stimulation. (m) The fluorescence intensity images of the four probes: PH-Akt-GFP, PBD-YFP, MLC-GFP and actin-GFP, in micropatterned MEFs without any cell–cell contact. (n) The bar graphs represent the polarity or intensity ratios between the free and junction end as described in Methods (mean±s.e.m., Student’st-test,**P<0.01).—PDGF: before PDGF;+PDGF: after PDGF stimulation. Norm., normalized. Scale bars, 10 μm. Figure 1: The polarization of molecular signals. MEFs transfected with various fluorescent probes were seeded on Fn-coated strips (10 μm in width), with one end free and the other end contacting a neighbouring cell. The broken white lines represent the body contours of neighbouring cells physically contacting the cells of interest. The hollow and filled arrows on the images indicate the positions of the free and junction ends, respectively. ( a – l ) The fluorescence intensity distributions of mCherry together with ( a – c ) PH-Akt-GFP ( n =4), ( d – f ) PBD-YFP ( n =5), ( g – i ) MLC-GFP ( n =4) or ( j – l ) actin-GFP ( n =4) before and after PDGF stimulation. ( a , d , g and j ) The pseudo colour images represent the fluorescence intensity of different probes as indicated, with cold and hot colours representing low and high fluorescence intensities, respectively; ( b , e , h and k ) The intensity distributions of indicated probes averaged along the strip direction before and after PDGF stimulation for various periods of time as indicated. ( c , f , i and l ) The averaged intensity ratios between the indicated probe and co-transfected mCherry along the strip direction before and after PDGF stimulation. ( m ) The fluorescence intensity images of the four probes: PH-Akt-GFP, PBD-YFP, MLC-GFP and actin-GFP, in micropatterned MEFs without any cell–cell contact. ( n ) The bar graphs represent the polarity or intensity ratios between the free and junction end as described in Methods (mean±s.e.m., Student’s t -test,** P <0.01).—PDGF: before PDGF;+PDGF: after PDGF stimulation. Norm., normalized. Scale bars, 10 μm. Full size image YFP-tagged p21 binding domain of p21-activated kinase (PAK-PBD-YFP) was used to localize active Rac [10] , [30] . As shown in Fig. 1d–f , active Rac monitored by PAK-PBD-YFP was concentrated at the free end before and after PDGF stimulation ( Supplementary Fig. S3b and Supplementary Movie 2 lower panel). Interestingly, MLC and AF visualized with GFP-tagged MLC (MLC-GFP) [31] and GFP-tagged β-actin (actin-GFP), respectively, were concentrated near the junction both before and after PDGF stimulation ( Fig. 1g–l , Supplementary Fig. S3c,d and Supplementary Movie 4 ), possibly promoting the junction stability [32] . In contrast, cells without a contacting neighbour were not polarized ( Fig. 1m and Supplementary Fig. S3e ). We conclude that cell–cell contacts regulate the polarized distribution of these signalling and cytoskeletal molecules/activities. To further quantify these asymmetric molecular distributions, we calculated the ratio of fluorescence intensities between the free and junctional ends (see the Methods section and Supplementary Fig. S2 ). The average ratios of PH-Akt-GFP at the front/rear significantly increased from 0.64 to 1.36 after PDGF stimulation, indicating that PI3K activity polarized towards the free end after PDGF stimulation. Meanwhile, the intensity ratio of PAK-PBD-YFP was 1.42 and 1.79 before and after PDGF stimulation, respectively. This result indicates that the free-end polarization of Rac activity does not require but slightly increases with PDGF. Further, MLC-GFP and actin-GFP had low ratio values before or after PDGF, suggesting that MLC and AF were concentrated proximal to the junction independent of PDGF. Additionally, the free end/junction intensity ratio values of all four signals (PI3K/Rac activities, and MLC/actin distributions) from individual cells were averaged from multiple frames within 5 min before, or during 20–30 min after PDGF stimulation. These temporally averaged free end/junction ratio values were compared with the measurements based on randomly selected individual time points. The results indicate that these two methods give very similar results ( Supplementary Fig. S4 ). This result is consistent with the relatively stable intracellular gradients observed after treatment with PDGF. To exclude the effect of cell morphology on these observations, cells were co-transfected with each one of the probes plus mCherry. The intensity of the probe and mCherry were determined and collectively smoothed in each individual cell with the moving average method. The ratio between the smoothed intensity curves of probe and mCherry was then calculated and averaged from multiple samples ( Fig. 1c ). These ratios (probe/mCherry) showed similar polarity as the corresponding curves before normalization, with PI3K and Rac higher at the free end, and MLC and F-actin enriched at the junctional end. The observed polarization is therefore not an artifact from cell shape or volume. As an additional set of controls, we also examined the dependence of the fluorescence probes on relevant molecular activities. The PDGF-induced PH-Akt-GFP accumulation at the free end was abolished by the PI3K inhibitor, LY294002, but not by the MLC kinase inhibitor, ML-7 ( Supplementary Fig. S5a and Supplementary Movie 3 ). Polarization of PAK-PBD-YFP was also significantly inhibited by LY294002 ( Supplementary Fig. S5b and Supplementary Movie 5 ), confirming that Rac is downstream of PI3K although LY294002 treatment caused cell contraction possibly due to the reduction of actin polymerization and membrane protrusion, as well as the destabilization of focal adhesions at the free end after the inhibition of PI3K/Rac activities [33] , [34] . PAK-PBD-YFP polarization was also blocked by dominant-negative Rac (RacN17), but not by ML-7 ( Supplementary Fig. S5b ). In contrast, ML-7, but not LY294002, blocked the polarization of MLC-GFP ( Supplementary Fig. S5c ). Cytochalasin D, but neither ML-7 nor LY294002, blocked the actin-GFP polarization ( Supplementary Fig. S5d ). These results support the specificity of the probes used in these studies, and suggest that PI 3-kinase/Rac and actin/myosin are regulated independently. N-cadherin regulates the polarity of Rac/PI3K and MLC/AF In fibroblasts, the major classical cadherin at cell–cell adherens junctions is N-cadherin [35] , [36] . We therefore asked whether N-cadherin regulates the observed polarities in this system. Knockdown of N-cadherin by siRNA (short interfering RNA) in MEFs inhibited polarization of both PI3K/Rac activities and MLC/AF ( Fig. 2a–d and Supplementary Fig. S6a,b ; quantified in Fig. 2e and Supplementary Fig. S6c ), although the physical cell–cell contact remained relatively intact ( Supplementary Fig. 7 ). In fact, following knockdown, PI3K and Rac activities were high at both the free and junction ends ( Fig. 2a ). These molecular signals were unpolarized in Chinese hamster ovary (CHO) cells lacking classic endogenous cadherins but repolairzed when N-cadherin was expressed [37] ( Supplementary Fig. S8 ). Thus, N-cadherin mediates the polarization of PI3K/Rac activities and MLC/AF distributions. In support of this notion, the N-cadherin-neutralizing antibody GC-4 ( [38] ) inhibited the polarization of these components ( Supplementary Fig. S9a ). 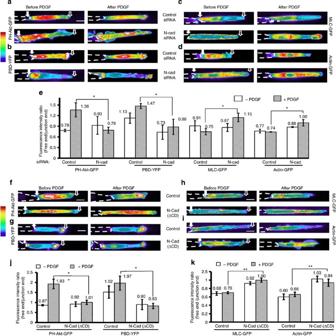Figure 2: N-cadherin mediates the polarity of PI3K/Rac activities and MLC/AF distributions. (a–d) MEFs were co-transfected with N-cadherin siRNA (50 nM) or control scramble siRNA (50 nM) together with the fluorescent probes (a) PH-Akt-GFP, (b) PBD-YFP, (c) MLC-GFP or (d) actin-GFP. The pseudo-coloured fluorescence intensity images showed the distributions of these probes in MEFs before and after PDGF stimulation. Representative images were selected generally within 20–40 min after PDGF stimulation. (e) The bar graphs represent different probe ratios (mean±s.e.m.,n=4, *P<0.05) of the fluorescence signal between the free and junction end of cell groups shown ina–d. (f–i) The intensity images of (f) PH-Akt-GFP, (g) PBD-YFP, (h) MLC-GFP or (i) actin-YFP before and after PDGF stimulation in MEFs transfected with or without N-cad(ΔCD). (j,k) The bar graphs (mean±s.e.m.,nfor each group was shown onSupplementary Fig. S11a–d, Student’st-test, *P<0.05 and **P<0.01) show the fluorescence intensity ratio (free/junction) of different probes in cell groups shown inf–gandh–i, respectively. The hollow and filled arrows on the images indicate the positions of the free and junction ends, respectively. Scale bars, 10 μm. Figure 2: N-cadherin mediates the polarity of PI3K/Rac activities and MLC/AF distributions. ( a – d ) MEFs were co-transfected with N-cadherin siRNA (50 nM) or control scramble siRNA (50 nM) together with the fluorescent probes ( a ) PH-Akt-GFP, ( b ) PBD-YFP, ( c ) MLC-GFP or ( d ) actin-GFP. The pseudo-coloured fluorescence intensity images showed the distributions of these probes in MEFs before and after PDGF stimulation. Representative images were selected generally within 20–40 min after PDGF stimulation. ( e ) The bar graphs represent different probe ratios (mean±s.e.m., n =4, * P <0.05) of the fluorescence signal between the free and junction end of cell groups shown in a – d . ( f – i ) The intensity images of ( f ) PH-Akt-GFP, ( g ) PBD-YFP, ( h ) MLC-GFP or ( i ) actin-YFP before and after PDGF stimulation in MEFs transfected with or without N-cad(ΔCD). ( j , k ) The bar graphs (mean±s.e.m., n for each group was shown on Supplementary Fig. S11a–d , Student’s t -test, * P <0.05 and ** P <0.01) show the fluorescence intensity ratio (free/junction) of different probes in cell groups shown in f – g and h – i , respectively. The hollow and filled arrows on the images indicate the positions of the free and junction ends, respectively. Scale bars, 10 μm. Full size image To identify the regions of N-cadherin required for the observed molecular polarization, we generated a series of N-cadherin dominant-negative mutants: N-Cad(ΔCD), N-Cad(Δp120), or N-Cad(Δβ-catenin), in which the entire cytoplasmic tail or the binding domain for either p120ctn or β-catenin was truncated ( Supplementary Fig. S9b ) [12] , [14] . Similar cadherin truncation mutants were previously used to dissect the cadherin/p120ctn and cadherin/β-catenin pathways [39] , [40] , [41] . The HA tag at the C-terminus of the cadherin mutants facilitates specific staining for the exogenous proteins ( Supplementary Fig. S9b ). Coimmunoprecipitation confirmed that N-Cad(ΔCD) failed to bind either p120ctn or β-catenin, whereas N-Cad(Δp120) or N-Cad(Δβ-catenin) had impaired binding of p120ctn or β-catenin only ( Supplementary Fig. S9c ). Nevertheless, N-Cad(ΔCD), N-Cad(Δp120) or N-Cad(Δβ-catenin), with their extracellular domains intact, still localized to cell–cell junctions ( Supplementary Fig. S9d ), although N-Cad(ΔCD) displayed less stability at junctions with altered morphology ( Supplementary Fig. S9d ). We further compared the distribution of the exogenous and endogenous N-cadherins, using HA antibody to recognize the exogenous N-cadherin or an N-cadherin antibody that reacts with the N-cadherin cytoplasmic domain. Thus, N-cad(ΔCD) can only be recognized by the HA antibody, while the endogenous N-cadherin only by the N-cadherin antibody. We observed that both exogenous N-cad(wt) and N-cad(ΔCD) localized at junctions, with N-cad(ΔCD) displacing the endogenous N-cadherin from junctions, as indicated by weaker junctional N-cadherin staining and certain suppression of endogenous N-cadherin expression level by exogenous N-cad(ΔCD) ( Supplementary Fig. S10 ). Immunostaining confirmed that N-Cad(Δp120) or N-Cad(Δβ-catenin) prevented the specific recruitment of endogenous p120ctn or β-catenin at junctions, respectively ( Supplementary Fig. S11a ). Therefore, the expression of exogenous N-cadherin mutants can dominantly suppress the localization/function of their endogenous counterparts. N-Cad(ΔCD), which does not bind p120ctn or β-catenin, clearly abolished polarization of both PI3K/Rac activities and MLC/AF distributions ( Fig. 2f–i ; quantified in Fig. 2j ). Interestingly, N-Cad(Δp120) only eliminated polarization of PI3K and Rac activities, resulting in activation at both ends of the cell, but without significant effect on MLC or AF ( Fig. 3a–d ; Supplementary Movies 6 and 7 ). In contrast, N-Cad(Δβ-catenin) blocked the polarity of MLC and AF, but not that of PI3K or Rac ( Fig. 3a–d and Supplementary Movie 8 ). These effects were confirmed by calculating the fluorescence ratios of free/junction ends ( Fig. 3e ) and the averaged curves of fluorescence signals along the strip directions ( Supplementary Fig. S12 ). Expression of N-Cad(Δp120) restored the polarity of MLC/AF but not that of PI3K/Rac activities in CHO cells ( Supplementary Fig. S13a ), whereas N-Cad(Δβ-catenin) restored the polarization of PI3K/Rac but not MLC/AF ( Supplementary Fig. S13b ). Thus, distinct regions of the N-cadherin cytoplasmic domain regulate different aspects of the molecular polarity in cells. 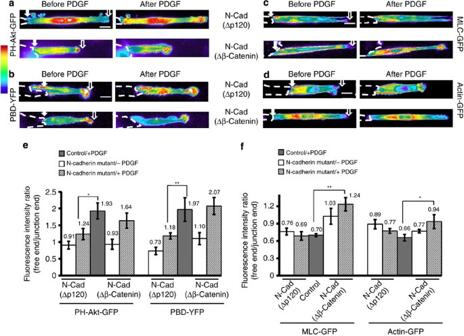Figure 3: P120ctn and β-catenin differentially regulate the polarity of PI3K/Rac and MLC/AF. The intensity images of (a) PH-Akt-GFP, (b) PBD-YFP, (c) MLC-GFP or (d) actin-YFP before and after PDGF stimulation in MEFs co-transfected with either N-cad(Δp120) or N-cad(Δβ-catenin) as indicated. (e,f) The bar graphs (mean±s.e.m.,nfor each group was shown onSupplementary Fig. S11a–d, Student’st-test, *P<0.05 and **P<0.01) represent the fluorescence intensity ratios (free/junction) of different probes in cell groups shown ina,bandc,d, respectively. The hollow and filled arrows on the images indicate the positions of the free and junction ends, respectively. Scale bars, 10 μm. Figure 3: P120ctn and β-catenin differentially regulate the polarity of PI3K/Rac and MLC/AF. The intensity images of ( a ) PH-Akt-GFP, ( b ) PBD-YFP, ( c ) MLC-GFP or ( d ) actin-YFP before and after PDGF stimulation in MEFs co-transfected with either N-cad(Δp120) or N-cad(Δβ-catenin) as indicated. ( e , f ) The bar graphs (mean±s.e.m., n for each group was shown on Supplementary Fig. S11a–d , Student’s t -test, * P <0.05 and ** P <0.01) represent the fluorescence intensity ratios (free/junction) of different probes in cell groups shown in a , b and c , d , respectively. The hollow and filled arrows on the images indicate the positions of the free and junction ends, respectively. Scale bars, 10 μm. Full size image The role of p120ctn and β-catenin The above results suggested that N-cadherin–p120ctn complexes may suppress junctional PI3K and Rac activities, whereas N-cadherin–β-catenin complexes promote the accumulation of MLC and AF near junctions. To further test these hypotheses, we expressed dominant-negative mutants of p120ctn and β-catenin [12] , [15] . P120(ΔARM1), a mutant of p120ctn that lacks the armadillo repeat necessary for binding to N-cadherin [15] , impaired the junctional localization of endogenous p120ctn, but not β-catenin ( Supplementary Fig. S11b ). This construct did not affect MLC or AF, but suppressed polarization of PI3K and Rac, leading to high activity at both ends ( Fig. 4a ). We also expressed β-catenin(Δα-catenin), which does not bind to α-catenin [12] or affect the junctional localization of p120ctn ( Supplementary Fig. S11b ). Consistent with the results of N-Cad(Δβ-catenin), β-catenin(Δα-catenin) abolished the polarity of MLC and AF, but not PI3K or Rac activity ( Fig. 4b ). Averaging fluorescence intensity along from multiple cells confirmed these effects ( Supplementary Fig. S14 ). We also examined a second β-catenin mutant, β-catenin(ΔN-cad) which does not bind to N-cadherin [42] . However, expression of this construct blocked N-cadherin localization and all the downstream functions ( Supplementary Fig. S15 ), possibly by suppressing the transcription and expression of N-cadherin [42] . Together, these results confirmed that the polarization of PI3K/Rac and MLC/AF is mediated by the N-cadherin–p120ctn and N-cadherin–β-catenin complexes, respectively. 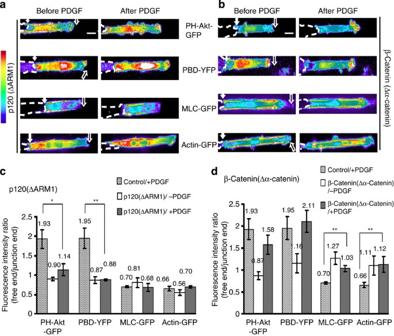Figure 4: The binding of p120ctn and β-catenin to N-cadherin regulates polarity. (a,b) The intensity images of the fluorescent probes PH-Akt-GFP, PBD-YFP, MLC-GFP or actin-GFP in MEFs co-transfected with (a) p120(ΔARM1) or (b) β-catenin(Δα-catenin). (c,d): The bar graphs (mean±s.e.m.,n=6, 5, 5, 6 for groups ofa, and 5, 6, 5, 6 for groups ofb, respectively. Student’st-test, *P<0.05 and **P<0.01) represent the fluorescence intensity ratios (free/junction) of different probes in cell groups shown inaandb, respectively. The hollow and filled arrows on the images indicate the positions of the free and junction ends, respectively. Scale bars, 10 μm. Figure 4: The binding of p120ctn and β-catenin to N-cadherin regulates polarity. ( a , b ) The intensity images of the fluorescent probes PH-Akt-GFP, PBD-YFP, MLC-GFP or actin-GFP in MEFs co-transfected with ( a ) p120(ΔARM1) or ( b ) β-catenin(Δα-catenin). ( c , d ): The bar graphs (mean±s.e.m., n =6, 5, 5, 6 for groups of a , and 5, 6, 5, 6 for groups of b , respectively. Student’s t -test, * P <0.05 and ** P <0.01) represent the fluorescence intensity ratios (free/junction) of different probes in cell groups shown in a and b , respectively. The hollow and filled arrows on the images indicate the positions of the free and junction ends, respectively. Scale bars, 10 μm. Full size image Integrin signalling mediates the polarity of PI3K and Rac activities Binding of integrins to their ligands can activate Rac [8] , [9] , [43] . We therefore examined the role of integrins in our system. GFP-conjugated integrin α5 was clearly polarized before and after PDGF stimulation, with a higher concentration at the free end ( Fig. 5a and Supplementary Movie 9 ). An antibody, 16G3, that binds Fn and blocks integrin binding [44] , completely inhibited the high PI3K and Rac activities at the free end, whereas the non-blocking Fn antibody 11E5 had no effect ( Fig. 5b ). 16G3, however, did not affect MLC or AF ( Fig. 5d ), suggesting that integrin signals specifically regulate PI3K and Rac. We also observed that Rac and PI3K activities were enhanced at the free end upon addition of MnCl 2 ( Supplementary Fig. S16 ), which directly activates integrins [45] . This result is consistent with the polarized integrin localization at the free end ( Fig. 5a ). Taken together, these data strongly suggest that integrins mediate the polarity of Rac and PI3K activities. 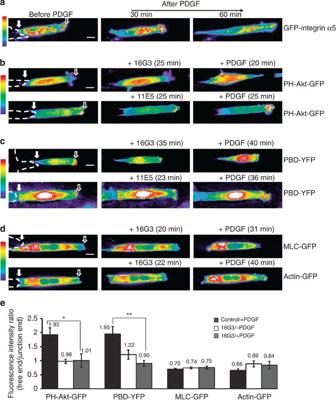Figure 5: Integrins mediate the polarity of PI3K and Rac activities. (a) The fluorescence intensity images of GFP-integrin α5 in a micropatterned MEF cell before and after PDGF stimulation. (b,c) The fluorescence intensity images of (b) PH-Akt-GFP or (c) PBD-YFP before and after the treatment with an Fn-blocking antibody 16G3 (+16G3) or a control non-blocking antibody 11E5 (+11E5) before the PDGF stimulation (+PDGF). (d) The fluorescence intensity images of the probe MLC-GFP or actin-GFP before and after the treatment with an Fn-blocking antibody 16G3 before the PDGF stimulation. (e) The bar graphs (mean±s.e.m.,n=4–6, Student’st-test, *P<0.05 and **P<0.01) show the fluorescence intensity ratios (free/junction) of the indicated probes with or without 16G3 pretreatment followed by PDGF stimulation. The hollow and filled arrows on the images indicate the positions of the free and junction ends, respectively. Scale bars, 10 μm. Figure 5: Integrins mediate the polarity of PI3K and Rac activities. ( a ) The fluorescence intensity images of GFP-integrin α5 in a micropatterned MEF cell before and after PDGF stimulation. ( b , c ) The fluorescence intensity images of ( b ) PH-Akt-GFP or ( c ) PBD-YFP before and after the treatment with an Fn-blocking antibody 16G3 (+16G3) or a control non-blocking antibody 11E5 (+11E5) before the PDGF stimulation (+PDGF). ( d ) The fluorescence intensity images of the probe MLC-GFP or actin-GFP before and after the treatment with an Fn-blocking antibody 16G3 before the PDGF stimulation. ( e ) The bar graphs (mean±s.e.m., n =4–6, Student’s t -test, * P <0.05 and ** P <0.01) show the fluorescence intensity ratios (free/junction) of the indicated probes with or without 16G3 pretreatment followed by PDGF stimulation. The hollow and filled arrows on the images indicate the positions of the free and junction ends, respectively. Scale bars, 10 μm. Full size image As integrins accumulate at the free end before PDGF stimulation ( Fig. 5a ) whereas the polarization of PI3K activity occurred mostly after PDGF ( Fig. 1a–c ), the polarity of PI3K activity may require the synergistic action of PDGFR and integrins. Interestingly, PDGFR also accumulated at the free end only after PDGF stimulation ( Supplementary Fig. S17a ). The polarized Rac activity in the absence of PDGF, on the contrary, may be directly promoted by the dynamic integrin ligation at the free end ( Fig. 1d–f ). Indeed, basal Rac polarity was abolished by the Fn-blocking antibody 16G3, but not by the non-blocking antibody 11E5 ( Supplementary Fig. S17b ). These results suggest that the activation of PI3K at the free end requires both integrins and PDGFR, whereas Rac can have substantial basal activation by integrins only, which can be further augmented by PDGFR. The N-cadherin–p120ctn axis suppresses integrins at the junction We next asked whether the N-cadherin–p120ctn axis regulates integrins to control the polarization of PI3K/Rac activities. Knockdown of N-cadherin by siRNA or the expression of N-cad(ΔCD) resulted in the accumulation of GFP-integrin α5 at both the free and junction ends ( Fig. 6a ). Expression of N-cad(Δp120), but not N-cad(Δβ-catenin), also increased integrin α5 at junctions ( Fig. 6b and Supplementary Movie 10 ). These results suggest that the association of p120ctn with N-cadherin may suppress the activation or trafficking of α5 integrin at cell–cell junctions. Consistent with this idea, GFP-integrin α5 localized at junctions in cells expressing p120(ΔARM1), but not in cells expressing β-catenin(Δα-catenin) ( Fig. 6c ). The ratio of integrin α5 intensity between the free and junction ends and the averaged curves of integrin α5-GFP fluorescence signal along the cell length confirmed that N-cadherin siRNA, N-cad(ΔCD), N-cad(Δp120) or p120(ΔARM1) induced integrin α5 accumulation at junctions whereas N-cad(Δβ-catenin) and β-catenin(Δα-catenin) had no effect ( Fig. 6d and Supplementary Fig. S18 ). Multiple independent results therefore support the conclusion that N-cadherin coupling to p120ctn blocks integrin function near cell–cell junctions. 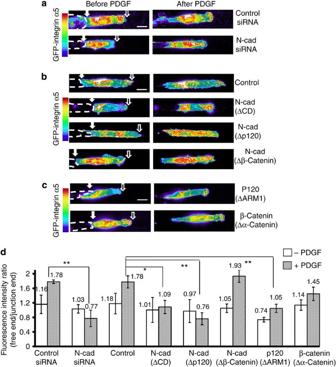Figure 6: The N-cadherin–p120ctn axis suppresses integrins at the junction. (a) The fluorescence intensity images of GFP-integrin α5 co-transfected with control siRNA (50 nM) (n=4) or N-cadherin siRNA (50 nM) (n=4) before and after PDGF stimulation. (b,c) The fluorescence intensity images of GFP-integrin α5 in cells co-transfected with empty control vector (n=5), N-cad(ΔCD) (n=5), N-cad(Δp120) (n=4), N-cad(Δβ-catenin) (n=4), p120(ΔARM1) (n=4) or β-catenin(Δα-catenin) (n=5) before and after PDGF stimulation. (d) The bar graphs (mean±s.e.m.,n=4 or 5, Student’st-test, *P<0.05 and **P<0.01) show the fluorescence intensity ratios (free/junction) of GFP-integrin α5 in MEFs under the conditions in (a–c). The hollow and filled arrows on the images indicate the positions of the free and junction ends, respectively. Scale bars, 10 μm. Figure 6: The N-cadherin–p120ctn axis suppresses integrins at the junction. ( a ) The fluorescence intensity images of GFP-integrin α5 co-transfected with control siRNA (50 nM) ( n =4) or N-cadherin siRNA (50 nM) ( n =4) before and after PDGF stimulation. ( b , c ) The fluorescence intensity images of GFP-integrin α5 in cells co-transfected with empty control vector ( n =5), N-cad(ΔCD) ( n =5), N-cad(Δp120) ( n =4), N-cad(Δβ-catenin) ( n =4), p120(ΔARM1) ( n =4) or β-catenin(Δα-catenin) ( n =5) before and after PDGF stimulation. ( d ) The bar graphs (mean±s.e.m., n =4 or 5, Student’s t -test, * P <0.05 and ** P <0.01) show the fluorescence intensity ratios (free/junction) of GFP-integrin α5 in MEFs under the conditions in ( a – c ). The hollow and filled arrows on the images indicate the positions of the free and junction ends, respectively. Scale bars, 10 μm. Full size image We then investigated whether integrin dynamics control the polarity of PI3K and Rac downstream of N-cadherin/p120ctn. The accumulation of PI3K activity at both the junction and the free end in cells expressing N-cad(Δp120) or p120(ΔARM1) was inhibited by 16G3, but not by 11E5 ( Fig. 7a ). Similarly, 16G3 blocked Rac activation at both ends in cells expressing N-cad(Δp120) or p120(ΔARM1) ( Fig. 7b ). These results confirmed that the N-cadherin–p120ctn axis suppresses integrins at the junction to inhibit PI3K and Rac. 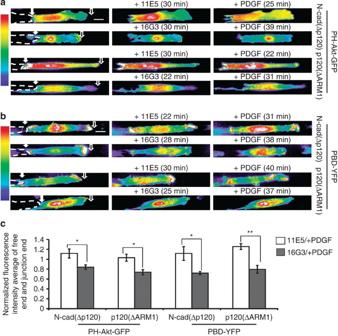Figure 7: The N-cadherin–p120ctn axis suppresses PI3K and Rac activities via integrins. The fluorescence intensity images of the probe (a) PH-Akt-GFP or (b) PBD-YFP in MEFs co-transfected with either N-cad(Δp120) or p120(ΔARM1) before and after the treatment with an Fn-blocking antibody 16G3 (+16G3) or a control non-blocking antibody 11E5 (+11E5) before the PDGF stimulation (+PDGF). (c) The bar graphs (mean±s.e.m.,n=4–6, Student’st-test, *P<0.05 and **P<0.01) show the normalized fluorescence intensity averages of free and junction ends of PH-Akt-GFP and PBD-YFP in MEFs after PDGF stimulation, with 11E5 or 16G3 pretreatment, for experiments shown inaandb(seen Methods for details of quantification). The hollow and filled arrows on the images indicate the positions of the free and junction ends, respectively. Scale bars, 10 μm. Figure 7: The N-cadherin–p120ctn axis suppresses PI3K and Rac activities via integrins. The fluorescence intensity images of the probe ( a ) PH-Akt-GFP or ( b ) PBD-YFP in MEFs co-transfected with either N-cad(Δp120) or p120(ΔARM1) before and after the treatment with an Fn-blocking antibody 16G3 (+16G3) or a control non-blocking antibody 11E5 (+11E5) before the PDGF stimulation (+PDGF). ( c ) The bar graphs (mean±s.e.m., n =4–6, Student’s t -test, * P <0.05 and ** P <0.01) show the normalized fluorescence intensity averages of free and junction ends of PH-Akt-GFP and PBD-YFP in MEFs after PDGF stimulation, with 11E5 or 16G3 pretreatment, for experiments shown in a and b (seen Methods for details of quantification). The hollow and filled arrows on the images indicate the positions of the free and junction ends, respectively. Scale bars, 10 μm. Full size image Subcellular polarity of signalling pathways is crucial for multiple cellular functions, including cell migration, tissue morphogenesis and cancer invasion [2] . To mimic collective cell migration in vivo , we established a model system, which avoids the damage of cells at the wounded edge and the subsequent release of chemical stimuli, as well as the debris remained in the wounded area. This model system also allows the convenient projection of molecular signals in one dimension, which facilitates statistical analysis and comparison among different cells. The ECM-coated strips constrain cell polarity movement to one dimension, thus facilitating analyses. Similar model systems utilizing micropatterning techniques have been successfully employed to demonstrate that the cell–cell adhesions can cause polarized cell morphology and centrosome distributions [18] , [19] . In this model system, the activities of PI3K and Rac concentrated at the free end of the cells, whereas MLC and AF accumulated near the junctional end. Polarity of PI3K and Rac depended on the N-cadherin–p120ctn complex, which acted by suppressing integrin function at the junctional end. By contrast, polarity of MLC and AF required the N-cadherin–β-catenin complex. These results therefore identify an integrated molecular network by which N-cadherin coordinates the subcellular polarity of different signalling molecules/activities through distinct effectors ( Fig. 8 ). 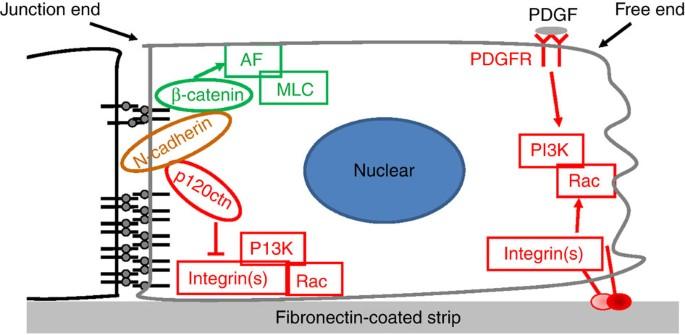Figure 8: Mechanism of adherens junction complex in regulating molecular polarity. A schematic diagram depicting the mechanism by which the N-cadherin–p120ctn and N-cadherin–β-catenin complexes differentially regulate the polarity of PI3K/Rac activities and MLC/AF distributions. Green indicates pathways that regulate MLC and AF; red indicates pathways that regulate PI3K and Rac. Figure 8: Mechanism of adherens junction complex in regulating molecular polarity. A schematic diagram depicting the mechanism by which the N-cadherin–p120ctn and N-cadherin–β-catenin complexes differentially regulate the polarity of PI3K/Rac activities and MLC/AF distributions. Green indicates pathways that regulate MLC and AF; red indicates pathways that regulate PI3K and Rac. Full size image Although E-cadherin is well known to induce PI3K/Rac activation during the formation of cell–cell junctions [46] , [47] , we found that stable N-cadherin junctions inhibited PI3K/Rac. This inhibitory effect of N-cadherin is consistent with previous reports [18] , [19] , [20] , [48] , [49] . We also found that the inhibition is mediated by local suppression of integrins through p120ctn. It has been reported that p120ctn can associate with E-cadherin to prevent the recruitment and activation of Rap1, which is an activator of the integrin functions [26] . Thus, the N-cadherin–p120ctn complex may also locally inhibit integrin activity through this pathway. Our data further suggest that high PI3K and Rac activities at the free end involve cooperation between integrins and PDGFR. Activated integrins have been shown to associate and co-localize with PDGFR at the leading edge of migrating cells and to promote PDGFR activation [50] . Consistent with these results, we found that integrin ligation specifically promoted PDGFR activation at the free end upon PDGF stimulation. Integrin ligation can also directly recruit and activate Rac at membrane lipid rafts [9] , [43] to mediate basal Rac activation and polarization. After addition of PDGF, integrins induce polarized activation of PDGFR, which recruits and activates PI3K to further activate Rac. Polarized integrin activity thereby appears to drive polarized Rac activation through both direct and indirect mechanisms. These ‘push and pull’ effects at the two ends of the cell hence result in the polarity of PI3K and Rac activities upon PDGF stimulation. MLC and AF concentrated at the two parallel edges near the junction. The arrangement of MLC depends on the acto-myosin contractility ( Supplementary Fig. S5 ) [51] , likely due to high Rho activity in this region [14] , [15] , [32] , [52] . Our results show that β-catenin bound to N-cadherin mediates this polarity. To what extent β-catenin physically anchors actin filaments at these sites through α-catenin or other linkers, as opposed to controlling Rho activity through guanine-nucleotide exchange factors or GAPs, remains to be determined. Immunofluorescence with an N-cadherin antibody against its cytosolic tail suggests that exogenous N-cad(ΔCD) expression in cells displaced endogenous N-cadherin from the junctions ( Supplementary Fig. S10 ). Expression of exogenous N-cadherin, p120ctn or β-catenin mutants specifically impaired the junctional localization of their target catenins but had minimal non-specific effect on other components ( Supplementary Fig. S11a,b ). Although the β-catenin-binding domain in the cytoplasmic tail of E-cadherin is reportedly important for functional cell–cell adhesion and junctional localization [53] , [54] , other cadherins behave differently. For N-cadherin, the lack of catenin-binding domain in the cytoplasmic tail does not prohibit the correct localization [40] . VE-cadherin with a truncated cytoplasmic tail also localized at cell–cell junctions [39] . Our results that N-cadherin mutants deficient in either p120 or β-catenin binding still localized to junctions ( Supplementary Figs S9d and S11a ) are therefore consistent with several previous reports. The contours of neighbouring cells physically contacting the cell of interest indicate that the knockdown of N-cadherin by siRNA or the expression of N-cadherin/catenin mutants did not significantly affect the contact areas among neighbouring MEFs on the micropatterned Fn strips. It is possible that the physical cell–cell contacts between neighbouring cells were maintained by other receptors such as JAMs or nectins despite impaired N-cadherin function, as cells were constrained on the Fn-coated strips. Therefore, our model system can allow the study of cadherin/catenin functions in regulating molecular polarity without the disruption of physical cell–cell contacts. In summary, our study presents evidence that cell–cell junctions determine the molecular polarity through a network of downstream effectors that independently control Rac and PI3K at the free edge, and actin and myosin at the junctional side. Surprisingly, the effect on Rac and PI3K is mediated by local control of integrins, which regulate both basal and PDGF-induced activities. These interlocking mechanisms are likely to determine collective cell migration in development, wound healing, cancer and other settings. Gene construction and DNA plasmids The complementary DNAs of N-cadherin and its truncated mutants were amplified from GFP-fused chicken N-cadherin construct [55] and fused with a HA tag (haemagglutinin epitope tag YPYDVPDYA) at the C-terminus by PCR before being cloned into pcDNA3.1 vector (Invitrogen) for mammalian cell expression ( Supplementary Fig. S8b ). The full-length N-cadherin cDNA or its mutant N-Cad(ΔCD) with the intracellular tail truncated (aa 1–759) was amplified by PCR with a sense primer containing a Not I site and a Kozak sequence 5′-GCCACC-3′ before the start codon of ATG, and a reverse primer containing the sequence coding a HA tag, a stop codon, and an Xba I site. For N-cad(Δp120) or N-cad(Δβ-catenin), two cDNA fragments of N-cadherin with amino-acid sequences 1–759 and 813–912, or 1–839 and 863–912 were amplified by PCR and fused together via a Sph I site, respectively. All these PCR products were then cloned into pcDNA3.1 using the Not I/ Xba I sites. The mouse full-length p120ctn and its mutant p120(ΔARM1) with the ARM1 domain (aa 358–400) truncated were both directly amplified by PCR from the retroviral constructs LZRS-mp120-1A and LZRS-mp120 1A(ΔARM1) [56] with a sense primer containing a EcoR I site, a Kozak sequence 5′-GCCACC-3′, and a reverse primer containing a sequence coding the c-Myc epitope tag (EQKLISEEDL), a stop codon and a Not I site. The PCR products were cloned into pcDNA3.1 vector using the EcoR I/ Not I sites. The cDNAs of β-catenin and its truncated mutant were amplified by PCR from a GFP-fused Xenopus β-catenin construct kindly provided by Dr Robert M. Kypta (MRC laboratory for Molecular Cell biology, University College, London) and fused with the c-Myc tag at the C-terminus before being cloned into pcDNA3.1 vector (Invitrogen). The full-length β-catenin cDNA (aa 1–781) was amplified by PCR with a sense primer containing a BamH I site and a Kozak sequence 5′-GCCACC-3′, and a reverse primer containing the sequence coding c-Myc tag, a stop codon, and an Not I site. For β-catenin(Δα-catenin), two cDNA fragments of β-catenin with amino-acid sequences 1–117 and 149–781 were amplified by PCR and fused together via a EcoR I site, respectively. To construct mCherry plasmid, mCherry cDNA was directly digested out from MT1-MMP-mCherry previously described [57] by using EcoR I/ Xho I sites and ligated back into pcDNA3.1 using the same digestion sites. The construct of PDGFR-GFP is a kind gift from Dr Hamid Band (Eppley Institute for Research in Cancer and Allied Diseases, University of Nebraska Medical Center). The constructs of PH-Akt-GFP, PAK-PBD-YFP and N-cadherin-GFP (GFP-fused chicken N-cadherin) were kindly provided by Drs Tamas Balla (National Institute of Child Health & Human Development, National Institutes of Health), Klaus Hahn (Department of Cell and Developmental Biology, University of North Carolina-Chapel Hill), and Andre Sobel (Institut National de la Santé et de la Recherche Médicale, Unité Mixte de Recherche, France). Microscope, image acquisition and analysis Cells expressing various exogenous proteins were starved in cell culture medium with 0.5% fetal bovine serum for 36–48 h before being passed on Fn-coated micropatterns generated atop cover-glass-bottom dishes (Cell E&G). During imaging, the cells were maintained in CO 2 -independent medium (Gibco BRL) without serum at 37 °C. Images were collected by a Zeiss axiovert inverted microscope equipped with × 40 objective and a cooled charge-coupled device camera (Cascade 512B; Photometrics) using the MetaFluor 6.2 software (Universal Imaging). The parameters of dichroic mirrors, excitation and emission filters for different fluorescent proteins were described previously [58] . Results were highly consistent among different cells, thus, 4–5 cells were analysed for each condition to provide sufficient data for statistical analysis. The polarized signals were highly stable at 20–40 min after PDGF stimulation, therefore randomly selected representative fluorescent images from this time period were used for the quantification of molecular polarity ( Fig. 1a–l and Supplementary Movies 2–4 ). For the images analysis and polarity measurement, we have developed an automatic and objective procedure to quantify the polarized localization of fluorescent probes relative to the junction end [59] . All the fluorescence images were background-subtracted before quantification. The cell shapes were detected by segmenting the fluorescence intensity images using the Otsu’s method [60] and converted into binary mask images with values outside the cell set to zero. To analyse the data from different cells in a uniform framework, the masks and corresponding cell images were rotated so that the micropatterned strips were oriented horizontally, with the junction localized at the left side of the cell ( Supplementary Fig. S2 ). The cell lengths were normalized to unity in the x direction (strip or horizontal direction). For each individual cell, the fluorescence intensity within the cell mask along the x direction was projected and averaged in the y direction (perpendicular to the strip direction), and the averaged intensity curve was normalized by the whole-cell intensity and plotted against the normalized distance to the junction end ( Supplementary Fig. S2 ). As such, the normalized intensity curves from different cells can be plotted within a uniform framework to allow the precise comparison between different groups. The averaged intensities in the x-direction from multiple cells with the same experimental condition were calculated and an average curve was then created using MATLAB function smooth (Mathworks; Natick, MA) by filtering with locally quadratic regression utilizing a moving window of size 5 ( Supplementary Fig. S3 ). The overall behaviour of each group of multiple cells can then be represented by one single curve. To quantify the polarity of the fluorescence distribution, individual normalized intensity curves were smoothed using a weighted average within a moving window of 10% cell length (implemented with the MATLAB function ‘smooth’ with the ‘rloess’ option and ‘span=0.1’) ( Supplementary Fig. S2c ). Then the ratios of maximum values on the smoothed curve near the free end (between 0.75 and 1) and the junction (between 0 and 0.25) for each individual cell were calculated. As there was a substantial pool of GFP-integrin α5 accumulated around perinuclear regions, possibly reflecting those stored in the endo/exocytosis recycling route before being transported to the plasma membrane, the maximum intensity values of GFP-integrin α5 were selected on the smooth curves between 0 and 0.1 near the junction and between 0.9 and 1 near the free end to reduce the noise originated from the perinuclear integrin pool. The mean and s.e.m. of the polarity ratio in each group were calculated for comparison and analysis. To quantify the ratio between the probe and mCherry, the intensity curves were calculated in individual cells and collectively smoothed among all cells with the moving average method as described above. The ratio between the smoothed curve of probe intensity and that of mCherry intensity was then calculated. To quantify the effect of FN antibodies 11E5 or 16G3 on the accumulation of PI3K or Rac1 activity at both the junction and the free end in cells expressing N-cad(Δp120) or p120(ΔARM1), as shown in Fig. 7 , the average of maximal values on the smoothed normalized intensity curves near the free end (between 0.9 and 1) and the junction (between 0 and 0.1) for each individual cell were calculated. Note individual intensity curves were already normalized by whole-cell intensity, so this measurement should be independent of the expression level of the fluorescence probe in each cell ( Supplementary Fig. S2 ). Statistics were analysed with the two-tailed Student’s t -test, with P -values less than 0.05 indicating significance. Cell culture and transfection Cell culture reagents were obtained from GIBCO BRL. MEFs (from ATCC), CHO cells and CHO cells expressing exogenous N-cadherin (N-CHO) were cultured in Dulbecco’s modified Eagle’s medium supplemented with 10% fetal bovine serum, 2 mM L -glutamine, 100 unit ml −1 penicillin, 100 μg ml −1 streptomycin and 1 mM sodium pyruvate in a humidified 95% air, 5% CO 2 incubator at 37 °C before experiments. Different DNA plasmids and siRNA were transfected into cells by using Lipofectamine 2,000 according to the manual protocol (Invitrogen). The co-transfection condition was optimized for MEFs, with 3 μg of DNA for each plasmid in each 35 mm cell culture dish. Reagents Recombinant rat PDGF-BB (50 ng ml −1 ) and MLC kinase inhibitor ML-7 (5 μM) were purchased from Sigma-Aldrich; PI3K inhibitor LY 294002 (10 μM) and Src inhibitor PP1 (10 μM) were purchased from Calbiochem and EMD Bioscience, respectively. ON-TARGETplus SMARTpool N-cadherin siRNA (N-cadherin siRNA) and ON-TARGETplus Non-Targeting siRNA (control siRNA) were purchased from Dharmacon RNAi technologies, Thermo Scientific. Anti-Fn antibodies 16G3 (20 μg ml −1 ) and 11E5 (20 μg ml −1 ) were previously described [44] . Mouse monoclonal p120 antibody, mouse monoclonal β-catenin antibody and mouse N-cadherin antibody were purchased from BD Transduction Laboratories. N-Cadherin-neutralizing antibody (GC-4) was from Sigma-Aldrich. Mouse monoclonal anti-HA antibody, rabbit anti-c-Myc and anti-HA antibodies, mouse anti-tubulin antibody and goat anti-NADPH antibody were from Santa Cruz Biotech. Goat FITC-conjugated anti-mouse and TRITC-conjugated anti-rabbit secondary antibodies were from Jackson ImmunoResearch. Methods for Micropatterning, Immunofluorescence, Immunoprecipitation (IP) and Immunoblotting (IB) can be found in the supplementary information . How to cite this article: Ouyang, M. et al. N-cadherin regulates spatially polarized signals through distinct p120ctn and β-catenin-dependent signalling pathways. Nat. Commun. 4:1589 doi: 10.1038/ncomms2560 (2013).